Delivery of therapeutic agents by nanoparticles made of grapefruit-derived lipids Although the use of nanotechnology for the delivery of a wide range of medical treatments has potential to reduce adverse effects associated with drug therapy, tissue-specific delivery remains challenging. Here we show that nanoparticles made of grapefruit-derived lipids, which we call grapefruit-derived nanovectors, can deliver chemotherapeutic agents, short interfering RNA, DNA expression vectors and proteins to different types of cells. We demonstrate the in vivo targeting specificity of grapefruit-derived nanovectors by co-delivering therapeutic agents with folic acid, which in turn leads to significantly increasing targeting efficiency to cells expressing folate receptors. The therapeutic potential of grapefruit-derived nanovectors was further demonstrated by enhancing the chemotherapeutic inhibition of tumour growth in two tumour animal models. Grapefruit-derived nanovectors are less toxic than nanoparticles made of synthetic lipids and, when injected intravenously into pregnant mice, do not pass the placental barrier, suggesting that they may be a useful tool for drug delivery. Nanotechnology is being applied to the area of drug delivery owing to the ability to deliver hydrophobic drugs and biologics, and preferentially target sites of disease [1] , [2] , [3] , [4] . However, despite these advantages for nanoparticle-based medicine delivery, it must overcome numerous obstacles including toxicity, the current cost of large-scale production and elimination of potential biohazards to the environment. Unlike the situation with nanoparticles synthesized artificially, nano-sized particles released from many different types of mammalian cells have been extensively studied recently [5] , [6] . Recently, nanoparticles released from mammalian cells have also been utilized for encapsulating drugs [7] and short interfering RNAs (siRNAs) [8] to treat disease in mouse models. Although this approach is promising, production of large quantities of mammalian cell nanoparticles and evaluation of their potential biohazards have been challenging [7] , [8] , [9] , [10] . In this study, nanoparticles are identified from the tissue of an edible fruit, grapefruit. In addition, a large quantity of nanoparticles is produced from grapefruit. Using in vitro cell culture models, as well as mouse tumour models, we have demonstrated that the grapefruit-derived nanovectors (GNVs) efficiently deliver a variety of therapeutic agents including chemotherapeutic drugs, DNA expression vectors, siRNA and proteins such as antibodies. Importantly, GNVs can be modified to achieve specific cellular targeting. This study demonstrates for the first time that GNVs are excellent candidates for delivery of a variety of different types of therapeutic agents. Characterization of GNVs Nanoparticles hold great promise as a therapeutic delivery vehicle; however, multiple parameters must be collectively optimized, including reducing/eliminating potential side effects, enhancing tissue- and cell-targeting specificity, and providing economical large-scale production. Making this process extremely difficult is the vast array of material and structural compositions that require analysis to fully optimize use of nanoparticles. We hypothesize that nanoparticles existing in edible plants would have limited to no toxicity to humans. Using standard techniques [11] , we first isolated particles from the juice of grapefruits. The particles from a sucrose gradient-purified band ( Fig. 1a , left panel) were identifiable as nanoparticles based on electron microscopic examination ( Fig. 1a , middle panel) and dynamic light scattering analysis (DLS, Fig. 1a , right panel). Nanoparticles purified from grape and tomatoes were also identified by electron microscopy and DLS (data not shown). Juices from edible plants are enriched for nanoparticles (1.76±0.15 g kg −1 of grape, 2.21±0.044 g kg −1 of grapefruit and 0.44±0.02 g kg −1 of tomatoes, means ±s.e.m. ), suggesting that certain edible plants could serve as a source for large-scale production of fruit-derived nanoparticles. 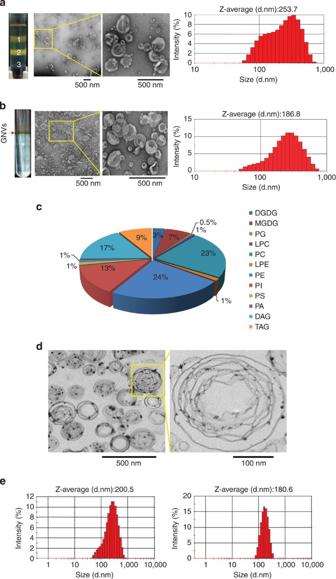Figure 1: Characterization of nano-sized particles made from grapefruit-derived lipids. (a) Sucrose-banded particles from grapefruit juice (left) and EM visualization of nano-sized particles (middle). Size distribution of the particles was further analysed by Zetasizer Nano ZS (right). (b) Sucrose-banded grapefruit lipid-derived GNVs indicated by the arrow (left) were examined using EM and photographed (middle). Size distribution of the particles was further analysed using a Zeta potential analyser (right). (c) Pie chart with a summary of the putative lipid species in GNVs, reported as percentage of total GNVs lipids. The composition is reported in detail inSupplementary Table S1in the Supporting Information. (d) GNVs embedded in polyBed 812 were sectioned and examined by electromicroscopy. Original magnification was × 50,000 (left) with enlargement of the indicated area shown in the right panel. (e) Size distribution of the GNVs before (left) and after (right) homogenization was further analysed using a Zeta potential analyser. Data (a,b,d,e) are representative of at least three independent experiments. Figure 1: Characterization of nano-sized particles made from grapefruit-derived lipids. ( a ) Sucrose-banded particles from grapefruit juice (left) and EM visualization of nano-sized particles (middle). Size distribution of the particles was further analysed by Zetasizer Nano ZS (right). ( b ) Sucrose-banded grapefruit lipid-derived GNVs indicated by the arrow (left) were examined using EM and photographed (middle). Size distribution of the particles was further analysed using a Zeta potential analyser (right). ( c ) Pie chart with a summary of the putative lipid species in GNVs, reported as percentage of total GNVs lipids. The composition is reported in detail in Supplementary Table S1 in the Supporting Information. ( d ) GNVs embedded in polyBed 812 were sectioned and examined by electromicroscopy. Original magnification was × 50,000 (left) with enlargement of the indicated area shown in the right panel. ( e ) Size distribution of the GNVs before (left) and after (right) homogenization was further analysed using a Zeta potential analyser. Data ( a , b , d , e ) are representative of at least three independent experiments. Full size image To determine whether lipids from grapefruit nanoparticles could be reassembled into nano-sized particles for use as a delivery vector, a standard method used for assembling liposomes was employed. Grapefruit nanoparticle-derived lipids were used for proof of concept and are referred to hereafter as GNVs. Based on electron microscopic examination ( Fig. 1b , middle panel) and DLS analysis ( Fig. 1b , right panel) of a sucrose gradient-purified band ( Fig. 1b , left panel) and the lipid profile ( Fig. 1c and Supplementary Table S1 ), the reassembled particles were nano sized. Electron microscopy results showed that most of the reassembled GNVs have a multilayer flower-like structure ( Fig. 1d ). Nanoparticles assembled from the lipids of two other sucrose gradient bands (band 1 and 3, Fig. 1a , left) were also prepared, and reproducibility for obtaining a single band of GNVs was somewhat unpredictable and sometimes double bands were formed ( Supplementary Fig. S1a ). In addition, the lipid profiles of band 1 and 3 were different from band 2 ( Supplementary Fig. S1b ). Although the GNVs generated initially from band 2 were heterogeneous in size, passing the GNVs through a homogenizer resulted in more uniform sized nanoparticles ( Fig. 1e ). Collectively, these results suggest that lipids derived from grapefruit nanoparticles can be reassembled into nano-sized particles and in large quantities. Tropisms and toxicity of GNVs To evaluate the potential use of GNVs as vectors to deliver therapeutic agents, the tropism and toxicity were evaluated. The efficient uptake of GNVs by different cell types was first evaluated. Each of the cell types was co-cultured with PKH26-labelled GNVs (PKH26–GNVs). The presence of GNVs in cells was examined using confocal microscopy ( Fig. 2a , top) or by fluorescence-activated cell sorting (FACS) ( Fig. 2a , bottom), and determined by quantitative analysis of PKH26–GNVs + cells. The results indicated that the majority of GL26, A549, SW620, CT26 and 4T1 cells internalized the GNVs. More than 20% of the B cells and 14% of the T cells took up the GNVs within 12 h of co-culture, which is remarkable as B and T cells are the most difficult to transfect using any commercially available transfection agents. When comparing the results with cells incubated with free PKH26 dye, distinct patterns of PKH26 + staining were observed in cells incubated with PKH26-labelled GNVs, which was not the case in cells incubated with free dye ( Supplementary Fig. S2 ). This suggests that the PKH26 + signals were derived from the GNV + cells, not from free PKH26 dye contamination. The results generated from A549, CT26, 4T1 and SW620 cells transfected with GNVs encapsulating psiCHECK 2 vectors further demonstrated that luciferase gene expressing vector, psiCHECK2, encapsulated by GNVs has biological activity upon entry into GNV-transfected cells ( Supplementary Fig. S3a ). Using A549 as an example, we further demonstrated that the efficiency of uptake of GNVs was a temperature-dependent process. Uptake rates were very slow at 4 °C and increased as the temperature was raised ( Fig. 2b ). The results from imaging ( Fig. 2b , top panel) or from FACS analysis ( Fig. 2b , bottom panel) of A549 cells co-cultured with PKH26-labelled GNVs indicated that >80% of A549 cells took up the GNVs at 37 °C but not at 20 °C or at 4 °C. Uptake of GNVs at 37 °C in the presence of the metabolic inhibitor sodium azide (50 mM) was significantly reduced after 3- and 6-h incubations ( Supplementary Fig. S3b ), suggesting that metabolic energy is required for this process. Under physiological temperature (37 °C) conditions, an initial rapid uptake of DiR dye-labelled GNVs (20 nmol ml −1 ) was observed within the first 2 h (the first time point) and was followed by a linear uptake that reached a peak between 12 to 24 h ( Fig. 2c ). The uptake of DiR dye-labelled GNVs by A549 cells was also found to be GNV concentration dependent. Treatment with the highest concentration (40 nmol ml −1 ) of GNVs resulted in no reduction of GNV uptake ( Fig. 2d ), suggesting that epithelial A549 cells have a high capacity for taking up GNVs. To further examine the mechanism of GNV internalization, A549 cells were treated with endocytosis inhibitors. Uptake of PKH26–GNVs ( Fig. 2e ) was markedly inhibited by the macrolide antibiotic bafilomycin A1, which prevents maturation of autophagic vacuoles. In addition, uptake of PKH26–GNVs was greatly diminished by treatment of A549 cells with cytochalasin D, an inhibitor of microfilament formation required for phagocytosis, nocodazole, an inhibitor of the polymerization of microtubules, and the clathrin-mediated endocytosis inhibitor chlorpromazine. Amiloride, an inhibitor of macropinocytosis, and the caveolae-mediated endocytosis inhibitor indomethacin did not affect uptake of PKH26–GNVs. Increasing the pH from 6.5 to 9.0 had no apparent effect on the uptake of GNVs ( Supplementary Fig. S3c ). We next sought to determine whether GNVs were toxic to A549 or CT26 cells. A cationic liposomes-DOTAP:DOPE (50/50) ( Supplementary Fig. S4 ) was used as a standard control. The results of uptake efficiency of GNVs and DOTAP:DOPE liposomes indicated that only about 40% of the cationic liposomes were taken up, whereas, more than 80% of GNVs was taken up ( Supplementary Fig. S5a ). The results of the ATPlite assay, which quantitatively measures cell proliferation, and the PI/Annexin V assay, which quantifies cell death, revealed that GNV treatment at concentrations up to 200 nmol ml −1 has no significant effect on A549 ( Supplementary Fig. S5b , top) and CT26 cell proliferation ( Supplementary Fig. S5b ) or the death rate of A549 cells ( Supplementary Fig. S5c ) in contrast with cells treated with cationic DOTAP:DOPE liposomes ( Supplementary Fig. S5 ). Furthermore, more than five passages of GNV-treated cells did not result in a reduction of cell doubling time when compared with the results of PBS-treated cells ( Supplementary Fig. S5d ). Collectively, these findings suggest that under physiological temperature conditions, GNVs are functionally taken up by both cell lines, as well as primary lymphocytes without cytotoxicity. Moreover, GNVs are much more stable than cationic DOTAP:DOPE liposomes at 37 °C in the presence of 10% bovine serum ( Fig. 2f ). In addition, GNVs were very stable at 4 °C for more than 1 month and did not lose their ability to carry curcumin, and maintained the biological activity of curcumin as determined by its inhibition of LPS-mediated induction of tumour-necrosis factor-α and interleukin-6 ( Supplementary Fig. S6 ). Based on the above results, GNVs have the capacity to deliver therapeutic products in vitro . 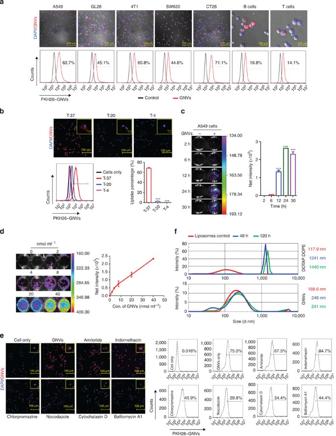Figure 2: Both hematopoietic and non-hematopoietic cells take up GNVs. (a) Confocal images (top) mouse and FACS quantitative analysis (bottom) of PKH26-labelled GNVs taken up by non-hematopoietic cells (A549, GL26, 4T1, SW620 and CT26) and primary splenic lymphocytes (T and B cells). (b) Temperature (T), (c) time (n=3) and (d) concentration dependence on the efficiency of GNVs uptake (n=3). (e) Potential pathways utilized by GNVs to enter A549 cells. (f) Stability of cationic DOTAP:DOPE liposomes (top) and GNVs (bottom) at 37 °C in the presence of 10% FBS. ***P<0.001 (Student’st-test). Data (a–e) are the mean±s.e.m. of at least five independent experiments. Figure 2: Both hematopoietic and non-hematopoietic cells take up GNVs. ( a ) Confocal images (top) mouse and FACS quantitative analysis (bottom) of PKH26-labelled GNVs taken up by non-hematopoietic cells (A549, GL26, 4T1, SW620 and CT26) and primary splenic lymphocytes (T and B cells). ( b ) Temperature (T), ( c ) time ( n =3) and ( d ) concentration dependence on the efficiency of GNVs uptake ( n =3). ( e ) Potential pathways utilized by GNVs to enter A549 cells. ( f ) Stability of cationic DOTAP:DOPE liposomes (top) and GNVs (bottom) at 37 °C in the presence of 10% FBS. *** P <0.001 (Student’s t -test). Data ( a – e ) are the mean±s.e.m. of at least five independent experiments. Full size image To determine the tissue tropism of GNVs, in vivo biodistribution of DiR-labelled GNVs was evaluated in mice using a Kodak Image Station 4000MM Pro system or the Odyssey imaging system. For these studies, we first evaluated the effect of different routes of injection on distribution of DiR-labelled GNVs. At 72 h after a tail-vein or intraperitoneal injection, DiR fluorescent signals were predominantly detected in the liver, lung, kidney and splenic tissues ( Fig. 3a ); whereas intramuscular injections of the DiR-labelled GNVs were predominantly localized in the muscle. After intranasal administration ( Supplementary Fig. S7 ) of DiR-labelled GNVs, the majority of the GNVs were located in the lung and brain. The presence and intensity of the imaging signal further indicated that DiR-labelled GNVs remain stable in the brain; whereas, no signal was detected in lung tissue 72 h after intranasal administration. FACS analysis was done on cells from mice receiving an intravenous (i.v.) injection of DiR-labelled GNVs. FACS analysis indicated that 72 h after GNVs were i.v. injected, they were taken up by splenic DX5 + NK cells (10.9%) and F4/80 + cells (12.5%), and liver F4/80 + cells (4.65%), DX5 + NK (1.75%) and CD19 + B cells (1.63%) ( Supplementary Fig. S8 ). Upon analysis of the stability of i.v.-injected DiR-labelled GNVs, we found that the fluorescent signals remained strong without a significant decrease in the liver, spleen and lung while the signals decreased significantly in the kidney at day 1 and in the brain at day 5 ( Fig. 3b ). In vivo imaging to continuously track the stability of injected DiR-labelled GNVs further revealed that fluorescent signals remained strong in the liver and spleen at day 20 ( Fig. 3b ). Surprisingly, circulating DiR-labelled GNVs were still detectable 7 days after a tail-vein injection ( Fig. 3c ) and most of the GNVs were free particles in plasma; few particles were associated with blood cells ( Supplementary Fig. S9 ). More importantly, unlike artificial nanoparticles that cross the placental barrier in pregnant mice and cause pregnancy complications [12] , [13] , our in vivo imaging analysis shows that mice tail-vein injected with DiR-labelled GNVs seem to have no GNVs that pass through the placenta ( Fig. 3d ), suggesting that GNVs could be potentially used as a delivery vehicle for certain drugs in pregnant women. 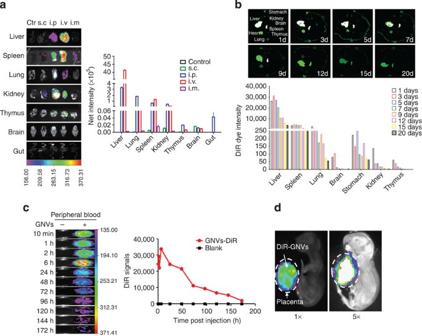Figure 3:In vitroandin vivostability and biodistribution of GNVs. (a) Biodistribution of DiR dye-labelled GNVs administrated subcutaneously (s.c.), intraperitoneally (i.p.), i.v. and intramuscularly (i.m.) to mice. (b)In vivostability of DiR dye-labelled GNVs was determined by scanning (Odyssey scanner) each organ of mice that received an i.v. injection of DiR-labelled GNVs. (c)In vivostability of circulating GNVs was determined by scanning (Kodak Image station) peripheral blood of mice injected i.v. with DiR dye-labelled GNVs. (d) Pregnant mice were injected i.v. with DiR dye-labelled GNVs 1 (1 × , left) or 5 times (5 × , right), the DiR signals (arrow indicated) in fetus and placenta (circled dotted line) were detected using a Kodak Image Station. (a–d) A representative image from each group of mice is shown, and followed by graphical figures presented as the mean net intensity (sum intensity/area,n=5). Data are representative of at least five independent experiments. Figure 3: In vitro and in vivo stability and biodistribution of GNVs. ( a ) Biodistribution of DiR dye-labelled GNVs administrated subcutaneously (s.c.), intraperitoneally (i.p. ), i.v. and intramuscularly (i.m.) to mice. ( b ) In vivo stability of DiR dye-labelled GNVs was determined by scanning (Odyssey scanner) each organ of mice that received an i.v. injection of DiR-labelled GNVs. ( c ) In vivo stability of circulating GNVs was determined by scanning (Kodak Image station) peripheral blood of mice injected i.v. with DiR dye-labelled GNVs. ( d ) Pregnant mice were injected i.v. with DiR dye-labelled GNVs 1 (1 × , left) or 5 times (5 × , right), the DiR signals (arrow indicated) in fetus and placenta (circled dotted line) were detected using a Kodak Image Station. ( a – d ) A representative image from each group of mice is shown, and followed by graphical figures presented as the mean net intensity (sum intensity/area, n =5). Data are representative of at least five independent experiments. Full size image To further explore the potential in vivo cytotoxic effects of the GNVs, proinflamamtory cytokines and indicators of liver injury were quantitatively determined. Serum levels of alanine aminotransferase and aspartate aminotransferase of mice pretreated with GNVs or DOTAP:DOPE liposomes were measured for liver injury. Alanine aminotransferase and aspartate aminotransferase were significantly increased after mice were treated with liposomes but not GNVs at a dose of 50 nmol per mouse or above ( Supplementary Fig. S10a ). Pro-inflammatory cytokines ( Supplementary Fig. S10b ) were not induced due to GNVs or DOTAP:DOPE liposome treatments. Histological analysis of tissues from GNV-treated animals ( Supplementary Fig. S10c ) revealed no pathological changes in the lung, kidney, liver or spleen when compared with tissues from untreated mice. Hepatocytes in the liver samples appeared normal, and there were no signs of an inflammatory response. No pulmonary fibrosis was detected in the lung samples. Necrosis was not found in any of the histological samples analysed. GNVs are candidate delivery vectors for therapeutics The molecular or drug therapy fields are currently limited by the lack of vehicles that permit high-efficiency transfection of targeted cells without a resulting cytotoxicity or host immune response. Our results ( Fig. 2 and Supplementary Fig. S5a ) demonstrate that GNVs were taken up in a highly efficient manner by a number of different types of cells without causing cytotoxicity or inducing an inflammatory cytokine response. Next, we determined whether the GNVs can deliver a broad range of therapeutic agents, such as chemotherapeutic drugs, siRNA, a DNA expression vector and proteins, to targeted cells. Our previously published data suggest that nano-sized particles released from mammalian cells favour binding to hydrophobic agents, such as curcumin and anti-stat3 JSI-124 (refs. 7 ), resulting in increased stability, solubility and bioavailability of these drugs. Results presented in this study also show that GNVs bind to hydrophobic agents including curcumin, folic acid (FA) and Zymosan A without altering the biological activities of the agents ( Supplementary Fig. S11 ). To further determine whether GNVs can also carry an agent that can serve as a conduit to deliver therapeutic agents, we chose biotin as a candidate as biotin is a small (244.31delta), hydrophobic molecule [14] . Biotinylated eYFP DNA expression vector carried by GNVs express the YFP protein in A549 cells as efficiently as those cells transfected with Lipofectamine 2000 ( Fig. 4a ). Furthermore, GNVs carrying biotinylized proteins like anti-CD4 or anti-CD8 antibodies significantly enhance the transfection efficiency of splenocyte CD4 + or CD8 + T cells ( Fig. 4b ), and the expression of the luciferase gene in these cells ( Fig. 4c ). This result suggests that GNVs encapsulating the luciferase gene carried in the psiCHECK 2 vector are internalized. Collectively, these results indicate that GNVs are capable of delivering both biotinylated DNA and proteins to targeted cells. 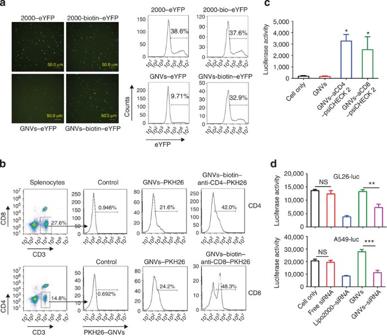Figure 4: GNV-mediated delivery of therapeutics. (a) A549 cells were transfected with biotinylated eYFP carried by GNVs or Lipofectamine 2000. A representative image of transfected cells is shown (left panel). YFP-positive cells were quantitatively analysed by FACS (right panel). (b) PKH26–GNVs loaded with biotin-labelled anti-CD4 or anti-CD8 antibodies were incubatedin vitrowith splenocytes and the PKH26-positive cells were qualitatively analysed by FACS. Data (a,b) are representative of at least three independent experiments. (c) GNVs-encapsulating psiCHECK2 were loaded with biotin-labelled anti-CD4 or CD8 antibodies, and then incubated with mouse spleen CD4+or CD8+cells. After 24 h, the expression of luciferase in CD4 and CD8 cells was detected. The results indicate the activity of luciferase expressed in the transfected T cells (n=5). (d) The biological effect of luciferase-specific siRNA carried by GNVs or Lipofectamine 2000 on inhibition of luciferase activity of transfected GL26-luc and A549-luc cells was evaluated using a luciferase assay (n=3). *P<0.05, **P<0.01 and ***P<0.001 (one-way analysis of variance, ANOVA). Data are the mean±s.e.m. of at least three independent experiments. Figure 4: GNV-mediated delivery of therapeutics. ( a ) A549 cells were transfected with biotinylated eYFP carried by GNVs or Lipofectamine 2000. A representative image of transfected cells is shown (left panel). YFP-positive cells were quantitatively analysed by FACS (right panel). ( b ) PKH26–GNVs loaded with biotin-labelled anti-CD4 or anti-CD8 antibodies were incubated in vitro with splenocytes and the PKH26-positive cells were qualitatively analysed by FACS. Data ( a , b ) are representative of at least three independent experiments. ( c ) GNVs-encapsulating psiCHECK2 were loaded with biotin-labelled anti-CD4 or CD8 antibodies, and then incubated with mouse spleen CD4 + or CD8 + cells. After 24 h, the expression of luciferase in CD4 and CD8 cells was detected. The results indicate the activity of luciferase expressed in the transfected T cells ( n =5). ( d ) The biological effect of luciferase-specific siRNA carried by GNVs or Lipofectamine 2000 on inhibition of luciferase activity of transfected GL26-luc and A549-luc cells was evaluated using a luciferase assay ( n =3). * P <0.05, ** P <0.01 and *** P <0.001 (one-way analysis of variance, ANOVA). Data are the mean±s.e.m. of at least three independent experiments. Full size image To determine whether GNVs would encapsulate and deliver functional siRNAs, we used a well-characterized siRNA that is directed against a luciferase reporter gene [15] stably expressed in GL26-Luc and A549-Luc. Transfection was conducted with 15 pmol luciferase siRNA delivered by GNVs or by a standard Lipofectamine 2000 transfection agent. We found that luciferase siRNA carried by GNVs effectively inhibited the expression of the luciferase gene when compared with GNVs alone or free luciferase siRNA-treated cells ( Fig. 4d ). In summary, the results show that GNVs are effective delivery vectors for all the agents we tested. In vivo targeting delivery of therapeutic agents with GNVs Previously, we showed [7] that the exosomes are capable of carrying the anti-Stat3 inhibitor, JSI-124, and that mice given an intranasal dose of nano-sized mammalian cell-derived exosomes carrying JSI-124 had a significant inhibition of GL26 tumour growth. We hypothesize that GNVs might also deliver JSI-124 to the brain via a non-invasive route and subsequently inhibit implanted GL26 tumour growth. In initial experiments, inhibition of Stat3 activity by GNVs–JSI-124 or JSI-124 was evaluated in 24-h cell cultures. Western blot assays revealed that JSI-124-loaded GNVs significantly inhibited the activation of Stat3 in comparison with GL26 tumours treated with GNVs only or PBS as controls ( Supplementary Fig. S12 ). Based on western blot results from cell cultures, groups of GL26 tumour-bearing mouse ( n =5) were intranasally administrated GNVs encapsulating the Stat3 inhibitor JSI-124 (12.5 pmol per 10 μl), GNVs only, JSI-124 only or PBS using an identical protocol as described previously [7] . Bioluminescent imaging of the mice treated as described above was used to quantify luciferase expression in relation to the GL26 tumour growth on days 5, 10, 15 and 20 post treatment. A representative image ( Fig. 5a , left panel) or imaging data ( Fig. 5a , right panel, top) showed the weakest luciferase expression that correlated to a reduction in tumour growth from the mice treated with GNVs encapsulating the Stat3 inhibitor JSI-124 compared with other groups. These results were further confirmed by the survival rates of mice. Survival of the PBS-, GNVs- or JSI-124-treated control animals ranged from 20 to 30 days. In contrast, GNVs–JSI-124 treatment significantly prolonged the survival of mice to an average of 42.5±2.3 days (mean±s.e.m.) ( Fig. 5a , right panel, bottom). 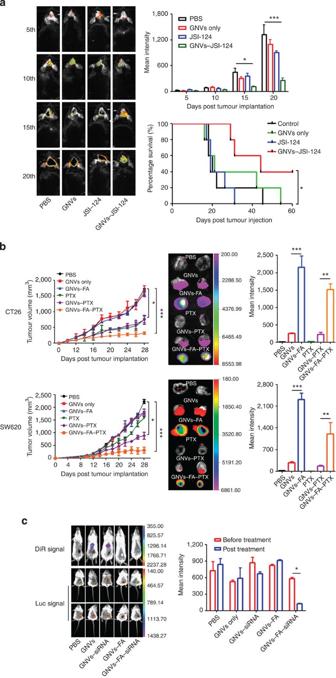Figure 5: Targeted delivery of GNVs carrying anti-cancer therapeutics. (a) C57BL/6J mice were implanted with GL26-Luc cells, GNVs were loaded with Stat3 inhibitor JSI-124 and then intranasally administrated to mice. The mice were imaged on post-injection days as indicated ina. A representative photograph showing the brain tumour signals of a mouse from each group (n=5) (a, left). The growth potential of injected GL26-Luc cells was determined by dividing photon emissions of mice treated with PBS by the photon emissions of mice treated with GNVs, JSI-124 or GNVs–JSI-124 (a, right, top). The results are based on two independent experiments with data pooled for mice in each experiment (n=5) and presented as the mean±s.e.m.; *P<0.05. Surviving percentage of GNVs–JSI-124-treated mice was compared with control mice. One representative experiment of two independent experiments is shown (n=5) (*P<0.05) (a, right, bottom). (b) Tumour cells were injected s.c. into BALB/c mice (CT26, 1 × 106per mouse, left, top) or NOD–SCID mice (SW620, 5 × 106per mouse, left, bottom). After tumour cells were injected, mice were treated with DiR dye-labelled agents as listed inFig. 5bvia i.v. injection every 3 days for a total of ten injections. Tumour volume was measured every 3 days. On day 30 after tumour cells were injected, tumours were removed and imaged with a Kodak Image station. Representative images of tumours from each group (n=5) are shown (b, middle). Right panels show the mean intensity of the DiR fluorescent signals of tumour (mean net intensity=sum intensity/area,n=5). The results are presented as the mean±s.e.m. **P<0.01 and ***P<0.001 (one-way and two-way analysis of variance, ANOVA). (c) CT26-Luc tumour cell-bearing mice were i.v. injected with luciferase siRNA (50 pmol per mouse in 200 nmol GNVs), luciferase siRNA carried by GNVs, or FA and luciferase siRNA co-delivered by GNVs every 3 days for a total of five injections. Representative images (left,n=5) and mean intensity of the luciferase activity of CT26-Luc tumour (right, mean net intensity=sum intensity/area,n=5) before and after treatments are presented. *P<0.05. Figure 5: Targeted delivery of GNVs carrying anti-cancer therapeutics. ( a ) C57BL/6J mice were implanted with GL26-Luc cells, GNVs were loaded with Stat3 inhibitor JSI-124 and then intranasally administrated to mice. The mice were imaged on post-injection days as indicated in a . A representative photograph showing the brain tumour signals of a mouse from each group ( n =5) ( a , left). The growth potential of injected GL26-Luc cells was determined by dividing photon emissions of mice treated with PBS by the photon emissions of mice treated with GNVs, JSI-124 or GNVs–JSI-124 ( a , right, top). The results are based on two independent experiments with data pooled for mice in each experiment ( n =5) and presented as the mean±s.e.m. ; * P <0.05. Surviving percentage of GNVs–JSI-124-treated mice was compared with control mice. One representative experiment of two independent experiments is shown ( n =5) (* P <0.05) ( a , right, bottom). ( b ) Tumour cells were injected s.c. into BALB/c mice (CT26, 1 × 10 6 per mouse, left, top) or NOD–SCID mice (SW620, 5 × 10 6 per mouse, left, bottom). After tumour cells were injected, mice were treated with DiR dye-labelled agents as listed in Fig. 5b via i.v. injection every 3 days for a total of ten injections. Tumour volume was measured every 3 days. On day 30 after tumour cells were injected, tumours were removed and imaged with a Kodak Image station. Representative images of tumours from each group ( n =5) are shown ( b , middle). Right panels show the mean intensity of the DiR fluorescent signals of tumour (mean net intensity=sum intensity/area, n =5). The results are presented as the mean±s.e.m. ** P <0.01 and *** P <0.001 (one-way and two-way analysis of variance, ANOVA). ( c ) CT26-Luc tumour cell-bearing mice were i.v. injected with luciferase siRNA (50 pmol per mouse in 200 nmol GNVs), luciferase siRNA carried by GNVs, or FA and luciferase siRNA co-delivered by GNVs every 3 days for a total of five injections. Representative images (left, n =5) and mean intensity of the luciferase activity of CT26-Luc tumour (right, mean net intensity=sum intensity/area, n =5) before and after treatments are presented. * P <0.05. Full size image In cancer therapy, accurate targeting of tumour tissue is required for successful therapy. Therefore, we tested whether GNVs can be modified to achieve tumour targeting. High-affinity folate receptors (FRs) are expressed at elevated levels on many human tumours and in almost negligible amounts on non-tumour cells [16] , [17] , [18] . Therefore, in this study, two tumour xenograft models including the mouse CT26 colon cancer model [19] and the human SW620 colon cancer SCID mouse model [18] were used to test whether GNVs binding FA would significantly enhance GNV targeting to tumour in a physiologic milieu. GNVs were labelled with DiR dye for in vivo imaging. At 72 h after i.v. injection of DiR dye-labelled GNVs, few DiR-labelled GNV signals were detected in tumour tissues with most signals being detected in the liver ( Supplementary Fig. S13 , second column from left). In contrast, i.v.-injected DiR-labelled GNVs–FA exhibited a much higher distribution to tumour tissues ( Supplementary Fig. S13 , third column from left). Co-delivery of FA with a chemotherapeutic drug (paclitaxel (PTX)) by GNVs has at least equal efficiency as GNVs–FA in targeting tumour tissue ( Supplementary Fig. S13 ), suggesting that co-delivery of FA with chemotherapeutic agents has no effect on FA-mediated targeting. Quantification of photons showed that DiR-labelled GNVs–FA distribution to tumour tissues was more than 1,300-fold (CT26 model) and 1,600-fold (SW620) greater than that of DiR-labelled GNVs ( Supplementary Fig. S13 , right panels). Next, we determined if co-delivery of FA with a therapeutic drug (PTX) by GNVs would have better therapeutic effect than the drug alone. As expected, the GNVs–FA–PTX treatment caused a substantial decrease in tumour growth in both tumour models. The tumour growth was significantly lower after treatment with GNVs–FA–PTX, an effect that was evident from day 20 (two tumour models) ( Fig. 5b , left panels). On day 30, the tumour volume in the PTX-loaded GNVs–FA group was 261.7±28.2 mm 3 , which was significantly smaller than that in other groups ( Supplementary Fig. S14 ). Consistent with the inhibition of tumour growth, FA carried by GNVs significantly enhanced the signals of DiR-labelled GNVs–FA or GNVs–FA–PTX in tumour tissues in both tumour models ( Fig. 5b , middle and right panels), indicating that the effect is attributable to the FA targeting the FR. In vivo biodistribution results on organs of killed tumour-bearing mice that were administered GNVs, GNVs–FA, PTX and GNVs–FA–PTX illustrated that free GNVs and PTX mainly targeted the liver and spleen, but FA- or FA–PTX-loaded GNVs primarily targeted tumours ( Supplementary Fig. S15 ). We further demonstrated that not only did GNVs–FA enhance the therapeutic effect of a chemotherapeutic drug by inhibiting implanted tumour growth, but it also dramatically enhanced the efficiency of delivery of siRNA to tumour. As shown in Fig. 5c , i.v. injection of GNVs–FA–siRNA–Luc led to more than a fivefold reduction in luciferase expression in CT26 tumour cells compared with GNVs–siRNA–Luc under the same conditions. Oral administration of GNVs as delivery vehicles has many advantages over other routes for therapy. Gut epithelial cells express several different FRs [20] , so we tested whether FA-conjugated GNVs enhanced GNV retention in the gut. Our results show that oral administration of GNVs–FA led to the enhancement of GNVs–FA signals in the stomach and small intestines of mice ( Supplementary Fig. S16 ). In this study, we hypothesize that edible plants may release nanoparticles that can be used in delivery of therapeutic agents. The results generated from examination of sucrose gradient-banded grapefruit-derived samples by electron microscopy and zeta potential indicates that there are nanoparticles released from the juice of grapefruit. Our findings have a number of advantages over currently existing technology as a delivery vehicle. A number of strategies, including nanotechnology and viral and non-viral delivery systems, have been used to experimentally determine the most suitable vector for treatment of diseases. Each of these approaches has advantages. However, potential toxicity, tissue-specific targeting, hazardous effects on the environment and large-scale economical production are challenging issues confronting these technologies [21] , [22] , [23] , [24] , [25] . Our approach using edible grapefruit-derived nanoparticles to make a nanovector has the advantage of having no detectable toxicity, the potential of being manipulated/modified for redirected targeting, the capacity to deliver a variety of agents and the ability to be produced economically. A simple and straightforward preparation process is required for practical large-scale generation of nanoparticles that can be loaded with multiple drugs. Our use of differential centrifugation followed by sonication allowed for large-scale production of GNVs. Our process is another major advantage over the multiple steps and cumbersome techniques required for in vitro synthesis of artificial or mammalian-based nanoparticles. Our results show that the GNVs created in this study can serve as the basis for developing more customized therapeutic delivery vehicles based on the disease. The incorporation of biotinylated therapeutic agents into a GNV considerably broadens the range of therapeutic agents and targeting moieties that could be delivered. The vector technology presented in this study as applied to cancer therapy could also be used for treatment of many other types of diseases by co-delivering therapeutic drugs with tissue-specific targeting agents. This study also demonstrated that chemotherapeutic drugs as well as siRNAs can be encapsulated into the nanovector and their biological effects in vivo are not altered. This is a crucial aspect for improving the delivery of siRNAs/miRNAs and chemotherapeutic drugs, especially, hydrophobic drugs. Stand-alone chemotherapy drugs suffer from numerous problems including rapid in vivo metabolism and/or excretion, an inability to access and penetrate cancer cells, and nonspecific uptake by healthy cells and tissues. Often a large percentage of a cytotoxic drug administered to a patient does not reach the tumour but is distributed throughout the body, causing the numerous toxic effects associated with chemotherapy thus reducing its therapeutic usefulness. In contrast, our GNVs are derived from edible plant tissue and is composed of biocompatible and biodegradable materials, encapsulates a wide range of drugs and drug classes, has the ability to attach in a targeting fashion to specific cell types or groups, protects the therapeutic agent from degradation and delivers the therapeutic agent directly to the site of disease. The size of a nanoparticle is a critical factor that prevents renal clearance (typically <20 nm), prevents uptake by the liver and spleen (particles >150 nm), and enhances accumulation in the tumour (particles between 50–150 nm) [26] , [27] , [28] , [29] . One advantage of the GNVs we developed is that the size can be further manipulated by changing the dispersity at which the nanovector passes through a high pressure homogenizer. This allows the vector size to be tailored for specific therapeutic treatments. We are now investigating the role of vector size on preferential accumulation of the vector in solid tumours via enhanced permeation and retention effects or other mechanisms [30] , [31] . An additional advantage of GNVs is its retention in the circulation for extended periods. Our data showed that the GNVs were detected on day 7 after i.v. injection. The longer the nanovector is in circulation, the more opportunity for the ERP effect and subsequent penetration into tumour tissues. The enhanced permeation and retention effect in combination with active targeting by the nanovector would enhance the therapeutic effect. Whether the GNVs in circulation at day 7 are more uniform in size and might favour retention of these GNVs in the blood needs to be further studied. In summary, we have shown that specially designed GNVs derived from edible nanoparticle lipids could shift the current paradigm of drug delivery using artificially synthesized nanoparticles to nanovectors derived from edible plants. Nanovectors derived from edible plants could be one of the safest therapeutic vectors because they do not cause cytotoxic reactions. Our demonstration of successfully inhibiting tumour growth in two independent murine cancer models using the GNVs suggests that it has potential for use as a delivery vehicle for treatment of various types of disease. Isolation and purification of grapefruit nanoparticles Grapefruits with the skin removed were manually pressed and the collected juice was diluted in PBS, differentially centrifuged (500 g for 10 min, 2,000 g for 20 min, 5,000 g for 30 min, 10,000 g for 1 h and 100,000 g for 2 h) and the nanoparticles then purified on a sucrose gradient [7] (8, 30, 45 and 60% sucrose in 20 mM Tris–Cl, pH 7.2). The purified nanoparticles were prepared for EM using a conventional procedure [32] and observed using an FEI Tecnai F20 electron microscope operated at 80 kV at a magnification of × 15,000 and defocus of 100 and 500 nm. Photomicrographs were taken using an AMT camera system. Assembling GNVs with lipids from grapefruit nanoparticles Total lipids were extracted from sucrose gradient band 2 ( Fig. 1 ) of processed grapefruit nanoparticles. Briefly, 3.75 ml 2:1 (v/v) MeOH:CHCl 3 was added to 1 ml of grapefruit nanoparticles in PBS and vortexed. CHCl 3 (1.25 ml) and ddH 2 O (1.25 ml) were added sequentially and vortexed. The mixture was centrifuged at 2,000 r.p.m. for 10 min at 22 °C in glass tubes to separate the mixture into two phases (aqueous phase and organic phase). For collection of the organic phase, a glass pipette was inserted through the aqueous phase with gentle positive pressure and the bottom phase (organic phase) was aspirated and dispensed into fresh glass tubes. The organic phase samples were aliquoted and dried by heating under nitrogen (2 psi). Total lipids were determined using the phosphate assay as described [33] . For assembling nano-sized particles (GNVs), residual chloroform was removed using a vacuum pump for 10–15 min and the dried lipids was immediately suspended in distilled water (150 ∼ 200 μl). After a bath sonication (FS60 bath sonicator, Fisher Scientific, Pittsburg, PA) for 5 min, an equal volume of buffer (308 mM NaCl, 40 mM Hepes, pH7.4) was added and sonicated for another 5 min. Before being used in experiments, the GNVs were homogenized by passing the samples through a high pressure homogenizer (Avestin Inc., Ottawa, Canada) using a protocol provided in the homogenizer instruction manual. Other protocols including labelling of GNVs and analysis of in vitro and in vivo trafficking of GNVs have been described previously [7] , [34] . Mice C57BL/6j mice, BALB/c mice and NOD/SCID mice 6–8 weeks of age were obtained from Jackson Laboratories. All animal procedures were approved by the University of Louisville Institutional Animal Care and Use Committee. Lipidomic analysis Lipid samples extracted from either grapefruit or GNVs were submitted to the Lipidomics Research Center, Kansas State University (Manhattan, KS) for analysis. In brief, the lipid composition of GNVs was determined by using a triple quadrupole mass spectrometer (an Applied Biosystems Q-TRAP, Applied Biosystems, Foster City, CA). The protocol has been previously described [35] . The data are reported as percentage of total signal for the molecular species determined after normalization of the signals to internal standards of the same lipid class. Confocal image analysis of localization of GNVs Tumour cells (4T1, GL26, A549, CT26 or SW620) were plated on four-chamber slides (Tissue-Tek, Sakura, USA) and cultured for 24 h at 37 °C. Then the cells were cultured with fresh culture media in the presence of PKH26-labelled GNVs (10 nmol ml −1 ). At variable time points after co-culture with PKH26-labelled GNVs, the cells were fixed with 2% paraformaldehyde in PBS for 20 min at 22 °C. The fixed cells were permeabilized with 0.2% Triton X-100 for 15 min and stained with 4′,6-diamidino-2-phenylindole (DAPI) for 90 s. PKH26-labelled GNVs in the cells were examined using a Nikon A1R-A1 confocal microscope equipped with a digital image analysis system (Pixera, San Diego, CA). For analysis of localization of GNVs in primary lymphocytes, freshly purified splenic T or B cells (5 × 10 6 ) were co-cultured with PKH26-labelled GNVs in a 24-well tissue culture plate for 6 h at 37 °C. After washing with PBS 3 × , the cells were fixed, permeabilized and stained with DAPI using the identical protocol as described above. Washed cells were centrifuged onto slides and PKH26-labelled GNVs in the cells were examined using a Nikon A1R-A1 confocal microscope equipped with a digital image analysis system (Pixera). To determine the effects of temperature on GNVs uptake, A549 cells were cultured in four-chamber slides at 37, 20 or 4 °C for 6 h with PKH26-labelled GNVs. After washing 3 × , GNVs-positive cells were observed using confocal microscopy. To study the effect of endocytosis inhibitors (amiloride 250 μM, indomethacin 100 μM, chlorpromazine 25 μM, nocodazole 25 μM, cytochalasin D 10 μM and bafilomycin A1 10 nM) on GNVs uptake, cells were cultured at 37 °C in the presence of an endocytosis inhibitor for 1 h before the addition of PKH26-labelled GNVs for an additional 6 h culture period. After washing with PBS 3 × , the cells were fixed with 2% paraformaldehyde in PBS for 20 min at 22 °C. The fixed cells were permeabilized with 0.2% Triton X-100 for 15 min and stained with DAPI for 90 s. Then the PKH26 + cells were visualized using confocal microscopy. Flow cytometry assay for uptake of grapefruit-derived GNVs For uptake experiments, tumour cells were grown in 12-well plates with Eagle’s minimal essential medium in the presence of 10% fetal bovine serum (FBS) for 24 h. PKH26-labelled GNVs (10 nmol ml −1 ) freshly prepared under sterile conditions were added to the culture media and incubated with cells for an additional 6 h. After washing with cold PBS 5 × , cells were trypsinized with 0.25% Trypsin-EDTA (Invitrogen) and washed an additional 2 × . Finally, the cells were resuspended in flow cytometry buffer and subjected to flow cytometry (BD Accuri C6 Cytometer, New Jersey, USA) and the results analysed using FlowJo Version 7.6 software (TreeStar Inc.). The data presented are based on the mean fluorescence signal for 50,000 cells collected. All assays were performed in triplicate. To study GNV taken up by primary lymphocytes, subsets of T and B cells were purified from the spleens of C57BL/6j mice with CD3 and CD19 beads, respectively (Miltenyl Biotec) according to the manufacturer’s protocol. In brief, spleens were removed aseptically and splenocytes were obtained by gently pressing the spleens between two sterile glass slides followed by washing the lymphocytes from the slides using 10 ml of RPMI 1640 medium containing 10% FBS. The cell suspension was pipetted several times and filtered through a 70-μm cell strainer (Falcon). The filtrate was then centrifuged at 1,200 r.p.m. for 5 min with 10% FCS–RPMI 1640 used for isolation of CD3 + T cells and CD19 + B cells according to the protocol provided (Miltenyl Biotec). Purified CD3 + T cells or CD19 + B cells were then resuspended and washed in RPMI 1640, cells were cultured in RPMI 1640 (Invitrogen) supplemented with 10% FBS, 2 mM L -glutamine, 100 U ml −1 penicillin, 100 μg ml −1 streptomycin, 25 mM Hepes, 50 μM 2-mercaptoethanol, 20 μg gentamicin and 1 mM sodium pyruvate in the presence of PKH26-labelled GNVs for 6 h at 37 °C in a 5% CO 2 incubator. The co-cultured cells were then washed with PBS 3 × . The percentage of PKH26 + cells was quantified by FACS analysis. To investigate the effect of pH on uptake efficiency, A549 cells (5 × 10 5 ) were seeded in 6-well plates and cultured for 24 h. The culture medium was replaced with fresh medium with different pH values (5.5, 6.5, 7.4 and 9.0) and cell culturing continued for 6 h with PKH26-labelled GNVs (10 nmol ml −1 ). The cultured cells were then washed with PBS 3 × . The percentage of PKH26 + cells was quantified by FACS analysis. To study the effect of endocytosis inhibitors on GNV uptake, cells were cultured at 37 °C in the presence of an endocytosis inhibitor for 1 h before the addition of PKH26-labelled GNVs, and culturing continued for an additional 6 h. The cultured cells were then washed with PBS 3 × . The percentage of PKH26 + cells was quantified by FACS analysis (BD Accuri Flow Cytometer) and FlowJo Version 7.6 software (TreeStar Inc.). To analyse the effects of temperature on GNV uptake, A549 cells were cultured in 6-well tissue culture plates with PKH26-loaded GNVs for 6 h at 37, 20 or 4 °C. After washing 3 × , PKH26 + cells were analysed using FACS. To determine whether the uptake of GNVs by A549 cells was energy dependent, confluent A549 cells were exposed to PKH26-labelled GNVs (10 nmol ml −1 ) for 3 and 6 h at 37 °C in the presence or absence of a metabolic inhibitor—50 mM sodium azide. After washing 3 × with PBS (pH7.4), PKH26 + cells were determined by FACS analysis as previously described [36] . Cells exposed to the vehicle (PBS; pH 7.4), served as a control. The data were analysed by FACS (BD Accuri TM Flow Cytometer) and FlowJo Version 7.6 software (TreeStar Inc.). To compare the uptake efficiency between GNVs and cationic liposomes-DOTAP:DOPE (50/50, w/w), A549 and CT26 cells (2 × 10 5 ) were incubated with the PKH26-labelled GNVs (10 nmol ml −1 ) or NBD-DOTAP:DOPE liposomes (10 nmol ml −1 ) for 3, 6 and 24 h at 37 °C. After 3 × washing with PBS, the percentage of PKH26 + cells or NBD + cells was determined by FACS analysis. To identify the cells that were targeted by GNVs in vivo , mice were i.v. injected with PKH26-labelled GNVs (200 nmol per mouse). At 72 h after injection, total spleen and liver cells resuspended in FACS analysis buffer were stained with anti-CD4, CD8, CD19, DX5 and F4/80 antibodies for further quantitative analysis of PKH26 + cells. Examining the ability of GNVs to cross the placental barrier To determine whether the GNVs passed through the placental barrier of pregnant mice and gain entry into the fetus, pregnant C57BL/6 mice were i.v. injected with DiR dye-labelled GNVs daily for 1 or 5 days (50 nmol injection per mouse, n =5). At 72 h after the last injection, the fetus and placenta were removed from anesthetized pregnant mice and imaged using the Odessey image system or a Kodak Image Station. Purification of drug-containing or dye-containing GNVs A chemotherapy drug, JSI-124, PTX or agents including FA, zymosan A or luciferase gene siRNA were mixed with total lipids from grapefruit dissolved in chloroform and dried under nitrogen to obtain a thin lipids-complex film. The film was reconstituted in PBS buffer, followed by sonication in a water bath sonicator for 30 min, allowing the lipids to self-assemble into drugs/chemicals/siRNA-loaded GNVs. The drug/chemicals/siRNA-loaded GNVs were purified using a sucrose gradient as described [11] . The purified band was collected and washed at 100,000 g for 2 h before use. For preparation and purification of GNVs loaded with biotin-labelled anti-CD4, CD8 antibodies, eYFP vectors or psiCHECK 2 vectors, biotin-labelled anti-CD4, CD8 antibodies (2.5 μg, BD Pharmingen, USA) were incubated with GNVs (200 nmol) at 4 °C overnight. The GNVs–biotin–anti-CD4 or GNVs–biotin–anti-CD8 complexes were washed with PBS at 36,000 r.p.m. for 2 h and the pellet was resuspended in PBS for the transfection of T cells. To prepare eYFP vector or psiCHECK 2 vector-loaded GNVs, biotin-labelled eYFP vectors (5 μg) or psiCHECK 2 vectors (3 μg) were incubated with GNVs (200 nmol) in OPTI-MEM for 2 h at 37 °C and subsequently used for transfection. Brain tumour-bearing mice model GL26-luc brain tumour-bearing mice were prepared as reported previously [7] . Tumour-bearing mice were treated intranasally for 10 consecutive days with GNVs, JSI-124 (12.5 pmol) or JSI-124-loaded GNVs. GL26 tumour growth was monitored by quantifying the activity of luciferase using a method as described [7] . Images were collected using a high-sensitivity CCD camera with wavelengths ranging from 300 to 600 nm with an exposure time for imaging of 2 min. Regions of interest were analysed for luciferase signals using the Kodak Image Station and reported in units of mean intensity. In vivo imaging of GNV-mediated targeting in tumour models Xenograft tumour growth models were used to demonstrate GNVs-mediated targeted delivery of chemotherapy drug to tumours versus standard chemotherapy with PTX. In our first set of experiments, 6-week-old female BALB/c mice (Jackson Laboratories) were injected subcutaneously with the murine colon cancer CT26 cell line (1.0 × 10 6 cells per mouse in 50 μl of PBS). In our second set of experiments, 6-week-old female NOD–SCID mice (Jackson Laboratories) were injected subcutaneously with the human colon cancer SW620 cell line (5.0 × 10 6 cells per mouse in 50 μl of PBS). When tumours reached ∼ 60 mm 3 in volume, the mice were randomly assigned to different treatment groups and injected i.v. with free GNVs, PTX (20 mg kg −1 of body weight), GNVs (200 nmol) loaded with FA (5 μg, GNVs–FA), GNVs (200 nmol) loaded with PTX (20 mg kg −1 of body weight, GNVs–PTX) and GNVs (200 nmol) loaded with FA plus PTX (GNVs–FA–PTX). Mice were treated every 3 days for 30 days with the last injection being DiR dye-labelled GNVs. Growth of the tumours was measured using a method as described [34] . Biodistribution of GNVs was monitored using a Kodak Image System after the final i.v. injection. Mice were killed, tumours and other organs were removed and biodistribution of DiR-labelled GNVs was analysed using a Kodak Image System. In vivo imaging of GNV-mediated siRNA delivery model CT26-luc tumour-bearing mice were prepared as described above and injected i.v. with free GNVs, FA-loaded GNVs, GNVs encapsulating the luciferase gene siRNA, or both FA and luciferase gene siRNA every 3 days for a total of five injections. Before starting the imaging, mice were intraperitoneally administrated D -luciferin (150 mg kg −1 ; Xenogen, Alameda, CA) dissolved in PBS and then anesthetized for determining the intensity of the mouse luciferase signals using a Kodak Image Station. Details of other methods used in this study are described in the Supplementary experimental procedures. Statistical analysis One-way, two-way analysis of variance (ANOVA) and t -test were used to determine statistical significance (* P <0.05, ** P <0.01 and *** P <0.001). How to cite this article: Wang, Q. et al . Delivery of therapeutic agents by nanoparticles made of grapefruit-derived lipids. Nat. Commun. 4:1867 doi: 10.1038/ncomms2886 (2013).